Genetic blueprint of the zoonotic pathogenToxocara canis Toxocara canis is a zoonotic parasite of major socioeconomic importance worldwide. In humans, this nematode causes disease (toxocariasis) mainly in the under-privileged communities in developed and developing countries. Although relatively well studied from clinical and epidemiological perspectives, to date, there has been no global investigation of the molecular biology of this parasite. Here we use next-generation sequencing to produce a draft genome and transcriptome of T. canis to support future biological and biotechnological investigations. This genome is 317 Mb in size, has a repeat content of 13.5% and encodes at least 18,596 protein-coding genes. We study transcription in a larval, as well as adult female and male stages, characterize the parasite’s gene-silencing machinery, explore molecules involved in development or host–parasite interactions and predict intervention targets. The draft genome of T. canis should provide a useful resource for future molecular studies of this and other, related parasites. Parasitic worms have a devastating, long-term impact on human health worldwide. For instance, approximately two billion people are infected with soil-transmitted helminths, such as hookworms ( Necator and Ancylostoma ), whipworm ( Trichuris ) and the large roundworm ( Ascaris ), principally in under-privileged areas of Latin America, Africa and Asia [1] . The global disease burden caused by these parasites is comparable with that of tuberculosis and malaria in disability-adjusted life years [1] . Ascaris , for example, infects more than one billion people, causing nutritional deficiency, impaired cognitive and physical development, principally in children and, in severe cases, death [2] . Published information [3] , [4] also shows that a related parasite, Toxocara canis (Werner, 1782), infects millions of people in poverty-stricken parts of the USA alone. Toxocariasis, the disease caused by Toxocara spp., is highly prevalent in many developing countries, where its importance is likely to be seriously underestimated. Toxocariasis results from zoonotic transmission of Toxocara spp. from carnivores, including canids and felids [5] , [6] . T. canis of canids is recognized as the main causative agent of zoonotic disease; this species has a complex life cycle, which can also involve paratenic hosts such as rodents. In humans, particularly children, T. canis larvae invade various tissues to cause visceral larva migrans, ocular larva migrans, neurotoxocariasis (including eosinophilic meningoencephalitis) and/or covert toxocariasis [7] . In addition, clinical and experimental studies [8] , [9] have indicated an association between T. canis infection and allergic disorders, such as asthma, chronic pruritus and urticaria. Both the canine and mouse models of T. canis [10] , [11] represent important tools for studies of the biology of the parasite, parasite–host interactions and toxocariasis at the immuno-molecular level. To facilitate such investigations, we sequenced and annotated the 317 Mb draft genome of T. canis and compare it with other nematode genomes. This genome contains at least 18,596 protein-coding genes, whose predicted products include at least 373 peptidases, 458 kinases, 408 phosphatases, 273 receptors and 530 transporters and channels. Notably, the T. canis secretome (870 molecules) is rich in peptidases proposed to be associated with the penetration and degradation of host tissues, and an assemblage of molecules suggested to modulate or suppress host-immune responses. This genome should provide a useful resource to the scientific community for a wide range of post-genomic studies of T. canis and could support the development of new interventions (drugs, vaccines and diagnostics) against toxocariasis and related nematodiases. 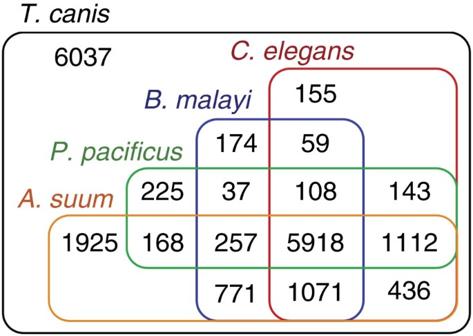Figure 1: Gene orthology. Venn diagram showing the number of orthologs betweenToxocara canisand four other nematode species,Ascaris suum,Brugia malayi,Caenorhabditis elegansandPristionchus pacificusupon pairwise comparison. Genome assembly and repeat content We sequenced the T. canis genome at 110-fold coverage and produced a final draft assembly of 317 Mb (N50=375 kb; Table 1 ) with a mean GC content of 40.0% (5.8% Ns). We detected 98.4% of the 248 core eukaryotic genes by Core Eukaryotic Genes Mapping Approach (CEGMA), indicating that the assembly represents a substantial proportion of the entire genome. We estimated a repeat content in this draft genome of 13.5% (equating to 42.9 Mb of DNA), comprising 1.8% DNA transposons, 4.1% retrotransposons, 1.4% unclassified dispersed elements and 6.4% simple repeats ( Supplementary Data 1 ); the overall repeat content is similar to that of the germline genome of the related worm Ascaris suum , but considerably higher than its somatic (diminuted) genome [12] , [13] . We identified 72,862 distinct retrotransposon sequences (see Supplementary Data 1 ) representing at least 68 families (16 LTR, 32 LINE and 20 SINE), with Gypsy , Pao and Copia predominating for LTRs ( n =12,436, 4,859 and 1,302, respectively) and CR1, RTE-RTEand L2 for non-LTRs ( n =16,073, 8,550 and 7,696, respectively). We also identified 61 families of DNA transposons (a total of 45,249 distinct sequences), of which CMC-EnSpm , Novosib and MULE-MuDR ( n =19,762, 2,787 and 2,501, respectively) predominated. This richness of families of transposable elements is comparable with that of genomes of other parasitic nematodes [12] , [14] , [15] . Table 1 Summary of the features of the Toxocara canis draft genome. Full size table The gene set of T. canis and comparison with other nematodes Using transcriptomic data from adult and larval stages of T. canis , de novo predictions and homology-based searching, we identified 18,596 coding genes, with mean gene, exon and intron lengths of 8,416, 156 and 1,133 bp, respectively, and an average of 7.4 exons per gene ( Table 1 ), similar to the findings for our Ascaris genome [12] . Compared with the draft genome sequences of A. suum [12] , [13] , Brugia malayi [14] , Caenorhabditis elegans [16] and Pristionchus pacificus [15] , on average, the T. canis genes have most sequence similarity to those of A. suum and are significantly longer than in the genomes of the other four nematodes, likely relating to an increased number and length of exons ( Supplementary Data 2 ). Most (67.5%) of the predicted T. canis genes ( Fig. 1 ) have an ortholog (BLASTp cut-off: 10 −5 ) in A. suum ( n =11,658; 62.7%), B. malayi (8,395; 45.1%), C. elegans (9,002; 48.4%) or P. pacificus (7,968; 42.8%). A total of 5,918 genes are orthologous among all 5 species, 3,557 are shared with at least 1 other species of nematode but absent from C. elegans and 1,925 are shared exclusively with Ascaris to the exclusion of the other 3 nematodes ( Fig. 1 ). Conversely, 6,037 genes (32.5%) are unique to T. canis relative to the other 4 nematodes ( Fig. 1 ). Of the entire T. canis gene set, 5,406 genes (29.1%) have an ortholog (≤10 −8 ) linked to known biological pathways (Kyoto Encyclopaedia of Genes and Genomes (KEGG); Supplementary Data 3 ). Mapping to pathways in C. elegans suggested a near complete complement of KEGG orthology groups (90.6%), also supporting the CEGMA results. By inference, most T. canis genes are represented in the present genomic assembly; at least 17,208 of all the 18,596 genes predicted here are supported by extensive transcriptomic and/or inferred proteomic data. Figure 1: Gene orthology. Venn diagram showing the number of orthologs between Toxocara canis and four other nematode species, Ascaris suum , Brugia malayi , Caenorhabditis elegans and Pristionchus pacificus upon pairwise comparison. Full size image Functional annotation and protein classifications In total, 14,583 (78.4%) of the protein sequences predicted from the 18,596 coding genes of T. canis were annotated based on the presence of characteristic protein domains ( Supplementary Data 4 ); 12,346 (66.4%) matches were found in C. elegans , and 10,977 (59.0%), 10,556 (56.8%) and 13,905 (74.8%) had significant matches in the InterProScan, Swiss-Prot and KEGG databases, respectively. Of the 10,977 InterPro matches, 9,121 (83.1%), 10,494 (95.6%), 1,827 (16.6%) and 412 (3.8%) were in Pfam, PANTHER, PRINTS and PIRSF databases, respectively. According to the KEGG BRITE hierarchy, predicted proteins represented peptidases ( n =373), kinases (458), phosphatases (408), receptors (273), transporters (530), GTPases (127), ion channels (268) and transcription factors (355); ( Supplementary Data 5 ), with some proteins inferred to have multiple functions. Key enzymes, channels, pore and transporters We identified five main classes of peptidases (metallo-, cysteine, serine, threonine and aspartic), with the metallo- ( n =165; 44.2%), cysteine (107; 28.7%) and serine (60; 16.1%) proteases predominating ( Supplementary Data 5 ). The most abundant families in these classes are the M12 astacins and adamalysins ( n =57), M01 aminopeptidases (19) and M13 neprilysins (13) among the metallo proteases; the C19 ubiquitin-specific proteases ( n =30), C01 papains (that is, cathepsins; 16) and C02 calpain-like enzymes (16) among the cysteine proteases; and the S01 ‘chymotrypsins’ ( n =12), S09 prolyl oligopeptidases (12) and S08 subtilisins (9) among the serine proteases. These secreted peptidases (for example, the M12 metallo, the C01 and C02 cysteine, as well as the S01, S08 and S09 serine proteases) are of major interest, given their presence in the excretory/secretory (ES) products of many parasitic helminths, and their central roles in tissue degradation and invasion (for example, during migration and/or feeding) and/or in immune evasion or modulation [17] , [18] . ES peptidases (including aminopeptidases and/or cysteine proteases) are likely to play key roles in these processes in T. canis and might represent important drug or vaccine targets. We also identified 458 protein kinases and 408 phosphatases in T. canis ( Supplementary Data 5 ). The kinome includes a large portion of serine/threonine protein (67.2%) and tyrosine (13.3%), as well as a small number of atypical or unclassified kinases (19.4%). The phosphatome includes predominantly serine-threonine (81.1%), protein tyrosine (12.7%) and a minority of other phosphatases. On the basis of the homology to molecules in the KEGG orthology (KO) database, we found 127 GTPases to be encoded in the T. canis genome, including 29 large (heterotrimeric) and 98 small (monomeric) G-proteins representing the Rab ( n =42), Ras (19), Arf/Sar (16), Rho (16) and Ran (1) families, as well as some unclassified molecules. Examples of these include C. elegans homologues eft-1 (gene Tcan_11808), fzo-1 (Tcan_14313), glo-1 (Tcan_03008) and rho-1 (for example, Tcan_13740; cf. Supplementary Data 5 ), which play essential roles in embryonic, larval and/or reproductive development and are also found in Ascaris [12] . Therefore, some of these enzymes might be targets for anti-parasite interventions. Also of interest in this context is the panel of channel, pore and transporter proteins that we identified here, particularly considering that many common anthelmintics bind representatives of some of these proteins as targets [19] . We predicted 156 GPCRs to be encoded in T. canis ; these include 111 class A rhodopsin family (for example, neuropeptide, serotonin, acetylcholine, dopamine and adrenaline receptors), 21 class B secretin receptor family (for example, parathyroid hormone, nematode chemoreception and latrophilin receptors), 10 class C metabotropic glutamate/pheromone family (for example, glutamate and gamma-aminobutyric acid (GABA) receptors) and 14 other (for example, Wnt) receptors ( Supplementary Data 5 ). In addition, of the 530 transporters predicted here, we identified an abundance of those of the solute carrier family (67.2%), major facilitator superfamily, ABC transporters (10.8%; including P-glycoproteins) and major facilitator superfamily (3.4%) [20] , [21] . In addition, we identified 268 ion-channel proteins ( Supplementary Data 5 ), the majority of which represented the Cys-loop superfamily (including nicotinic, glycine, aniononic and GABA-A; 39.6%), as well as voltage-gated cation (mainly K + channels, including SLO-1; 31.0%) and others related to voltage-gated cation channels (transient receptor potential; 10.8%), some of which are known targets for anthelmintic drugs [22] . Stage-, gut- and gender-enriched transcription profiles Here we defined clusters of genes that are significantly differentially transcribed between the T. canis adult and third-stage larvae (L3s from fully embryonated eggs), and between the two sexes of this nematode, by integrating data from KO enrichment, as well as co-transcription and functional network analyses ( Supplementary Data 6–9 ). In the T. canis life cycle, dioecious adults establish and live in the small intestine of the canid host following hepato-pulmonary migration of parasitic L3s [11] . By comparison to L3, we showed that pathways enriched in the adult stage involve carbon metabolism (for example, aldo-2 , c04c3. 3, enol-1 , fbp-1 , gpd-3 and gpi-1 ), lysosome activity, transport (ABC transporters), xenobiotic metabolism and DNA replication/repair, likely linked to digestive and reproductive processes in the worm ( Fig. 2 and Supplementary Data 4, 6 and 7 ). With reference to the adult stage, L3-enriched pathways were mostly linked to neuronal signalling (for example, ckr-2 , dop-1 , gar-2 and unc-49 ), and cuticle formation and/or shedding (including col-121 , dpy-5 and sqt-1 ; Fig. 2 and Supplementary Data 4, 6 and 7 ) which might relate to “fuzzy coat” shedding from L3s during immune attack in vitro [23] , [24] . Interestingly, homologues of various genes known to regulate dauer in C. elegans were upregulated (for example, daf-9 , daf-12 , osm-3 and osm-6 ) or downregulated (two paralogs of mek-2 ) in the L3 stage [25] , [26] ( Fig. 2 ), which supports the proposal that this stage is in an arrested state of development following the in vitro -hatching of embryonated eggs and maintenance in culture in the absence of host factors [24] . 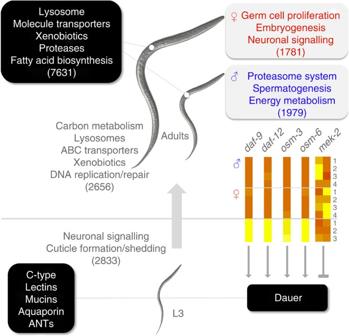Figure 2: Stage-, gut- and gender-enriched transcription. Key biological pathways or processes inToxocara canis, for which the gene transcription is enriched in adult females (red) and males (blue); in adults and third-stage larvae (L3; grey); and in the alimentary tract of the adult worms (black box, top left). Molecules enriched in L3s and involved in parasite–host interactions, such as immunomodulation, are also indicated (black box, bottom left; ANT, abundant new transcripts); the number of genes with significantly increased transcription are given in parentheses. The proposed arrested or dauer status of the L3 stage ofT. canis(from embryontated eggs) is supported by the transcription profiles (heat-map, right) for gene homologuesdaf-9,daf-12andosm-3,osm-6(upregulation; yellow) and twomek-2paralogs (downregulation; orange to red), which are all known to promote dauer inC. elegans; the biological replicates (1–4) studied are indicated to the right of the heat-map. Figure 2: Stage-, gut- and gender-enriched transcription. Key biological pathways or processes in Toxocara canis , for which the gene transcription is enriched in adult females (red) and males (blue); in adults and third-stage larvae (L3; grey); and in the alimentary tract of the adult worms (black box, top left). Molecules enriched in L3s and involved in parasite–host interactions, such as immunomodulation, are also indicated (black box, bottom left; ANT, abundant new transcripts); the number of genes with significantly increased transcription are given in parentheses. The proposed arrested or dauer status of the L3 stage of T. canis (from embryontated eggs) is supported by the transcription profiles (heat-map, right) for gene homologues daf-9 , daf-12 and osm-3 , osm-6 (upregulation; yellow) and two mek-2 paralogs (downregulation; orange to red), which are all known to promote dauer in C. elegans ; the biological replicates (1–4) studied are indicated to the right of the heat-map. Full size image In addition, in the worm, we showed that the intestinal tract of T. canis was specifically enriched for gene transcripts linked to molecular uptake and degradation via lysosomes (for example, vha-2 , -4 , -6 , -8 and -12 ), the transportation of amino acids, sugars, lipids and drugs, the metabolism of xenobiotic metabolism (for example, ugt-22 , -34 , -45 , -49 , -63 and cyp14a5 ), as well as protein digestion (aspartic, cysteine and metallo-peptidases) and fatty acid elongation (for example, elo-2 , -3 , -4 , -5 , -6 and -9 ; Fig. 2 and Supplementary Data 4, 6 and 7 ). These processes are consistent with extensive digestive, absorptive and detoxifying functions within the gut of T. canis and similar, in some respects, to those suggested for Ascaris [27] . Given the size of adult T. canis (usually 5–15 cm in length), we were able to investigate differential transcription between individual female and male worms. Genes with female-enriched transcription were linked to signal transduction pathways involving mainly neuroactive GABA glycine and acetycholine receptors, as well as G protein-coupled receptors associated with germ cell proliferation and embryogenesis ( Fig. 2 and Supplementary Data 4, 6 and 7 ). Female-enriched transcription related to genes encoding glycosyltransferases of N-acetyl glucose/galactosamine moieties linked to egg shell synthesis in oogenesis (for example, gene codes C36A4.4, F07A11.2 and F21D5.1), oocyte maturation and embryonic development (for example, ceh-13 , elt-3 , gsk-3 , kgb-1 , nrh-1 , pha-4 , rab-11.1 , unc-60, -130 and vab-2 ), egg laying (for example, lin-29 , nsy-1 , rhgf-1 , sem-2 and sox-2 ) and vulva development (for example , arf-1.2 , ceh-20 , let-23 , lin-1 and -61 ; Fig. 2 and Supplementary Data 4, 6 and 7 ). In contrast, genes with male-enriched transcription were inferred to be associated with protein degradation, spermatogenesis, epinephrine-like hormone regulation (tyramine and octopamine) and energy metabolism ( Fig. 2 and Supplementary Data 4, 6 and 7 ). Key genes with male-enriched profiles encoded proteasome-related enzyme groups as well as protein-serine/threonine and -tyrosine kinases linked to sperm and spermatogenesis. Conspicuous were those linked to the 26S proteasome and associated recycling of ubiquitin moieties (for example, pas-1 , rpn-1 , rps-26 , rtp-3 and rpt-5 ) involved in germline development and spermatogenesis (for example, cpb-1 , fog-3 and spe-6 ; Fig. 2 and Supplementary Data 4, 6 and 7 ). Overall, of all 3,760 genes exhibiting gender-enriched transcription, ~26% had no homologues in any other organisms for which genomic or transcriptomic data are publicly available. The secretome and molecules for parasite–host interactions We predicted the secretome of T. canis to comprise at least 870 ES proteins with a diverse array of functions ( Supplementary Data 10 ). Most notable are at least 14 peptidases, including 7 SC serine proteases (S1, S9 and S28 families), 3 aspartic proteases (A1 family), 3 CA/CD cysteine proteases (C1 and C13 families) and 1 MA metallo-protease (M14 family), as well as 23 cell-adhesion molecules (immunoglobulins, integrins and cadherins), 17 lectins (C-type) and 6 SCP/TAPS proteins (venom allergen homologues) [28] . Many secreted peptidases (representing the ‘degradome’) and their respective inhibitors have known roles in the penetration of tissue barriers and feeding by parasitic worms, including T. canis [5] , [23] . T. canis larvae invade various tissues, including muscles, brain and eyes, and cause clinical disease. Such larvae have an exceptional ability to evade or block host attack and can survive for many years in tissues. This ability is associated with the deployment of molecules excreted or secreted by the parasite or released from its surface coat [23] , [24] . Here, we predicted 33 proteins involved in host interactions and/or modulating host immune responses ( Supplementary Data 11 ). Abundant in O-linked glycosylations are mucins ( n =7), many of which are likely heavily targeted by IgM antibodies and bound by various pattern-recognition receptors associated with host dendritic cells, responsible for inducing a Th2 immune response [18] . Immunomodulatory molecules predicted in T. canis also include homologues (E-value cut-off=10 −8 ) of the B. malayi cystatin CPI-2 (B-cell inhibitor), several transforming growth factor-β and macrophage initiation-factor mimics, numerous neutrophil inhibitors, oxidoreductases, known to counteract the neutrophil oxidative burst, and five close homologues of platelet anti-inflammatory factor-α [18] . Key examples of T. canis ES proteins predicted to be involved in immune evasion include some ‘hidden’ antigens [29] (for example, numerous C-type lectins) with close homology to vertebrate macrophage mannose or CD23 (low affinity IgE) receptors, which mimic host molecules [18] . Other representatives include mucins (originating from the parasite’s surface coat), phosphatidylethanolamine-binding proteins, cathepsins, asparagyl endopeptidases (legumains), superoxide dismutases, SCP/TAPS [28] , olfactomedin, aquaporin, prohibitin and various orphan proteins (including abundant new transcripts (ANTs)), identified previously in small-scale molecular studies of T. canis [23] , [24] . Interestingly, although not encoded in the genome, ant s-3, -5, -30 and -34 were transcribed at very high levels in all tissues of one of four female T. canis studied here and at high levels in all L3 samples, but were transcribed at very low levels or not at all in tissues of the adult males ( Supplementary Data 11 ). Three-dimensional modelling of all predicted ANTs showed that ANT-5 is an RNA-dependent RNA polymerase and that ANT-34 is a RNA helicase, consistent with previous findings [30] . The absence of the ant genes from the draft genome, the similarity in the structures of ANT-5 and ANT-34 with viral proteins and the inconsistency in their transcription in stages, sexes and/or tissues of T. canis suggest that ant transcripts are derived from one or more double-stranded-RNA viruses. This proposal warrants investigation to establish whether ANTs are crucial to the biology of T. canis and indeed have a role in regulating transcription [30] . Overall, the present genomic and transcriptomic data sets reveal that, on a global scale, T. canis possesses a major arsenal of ES proteins that are involved in manipulating, blocking and/or evading immune responses in host animals. A detailed understanding the roles of these molecules could pave the way to new intervention strategies, such as vaccination. New intervention targets and molecular function Given that only a small number of drugs are effective against toxocariasis in accidental (human) or paratenic hosts [31] , there is a need for improved treatments. In particular, genomic-guided drug-target discovery provides an alternative means to conventional screening and re-purposing [32] . The goal of such discovery is to predict (essential) genes or gene products, whose inactivation by one or more drugs selectively kills the nematode but does not harm the mammalian host. Essentiality can be inferred from functional information (for example, lethality) in C. elegans [33] , [34] , and this approach has already yielded credible targets in nematodes [35] . Here, in T. canis , we predicted 715 essential orthologs, of which 703 were linked to lethal-gene knock-down phenotypes in C. elegans ( Supplementary Data 12 ), of which 230 had ligands that met the Lipinsky rule-of-five [36] , [37] ( Table 2 and Supplementary Data 12 ). Using stringent criteria, we identified eight channels or transporters (including GABA, acetylcholine receptors and SLO-1 calcium-activated potassium channels), already recognized as targets for various anthelmintics, including AADs, cyclic depsipeptides, imidazothiazole derivatives (including levamisole) or macrocyclic lactones [19] , [22] , [38] , [39] . Also notable are 57 kinases, 21 peptidases, 14 phosphatases (including PP1 and PP2A homologues, as specific targets for norcantharidin analogues) [40] , 5 GTPases and 4 GPCRs ( Table 2 ). The validity of these prioritized targets can now be tested on T. canis in vitro by gene silencing, and subsequently with drugs. Table 2 Druggable candidates represented in the Toxocara canis genome. Full size table Although stages of the parasite cannot be produced in culture, L3s of T. canis can be maintained in vitro in serum-free medium for extended periods (at least 18 months) [41] , suggesting that this stage might be amenable to gene silencing by double-stranded-RNA interference (RNAi) or using specific inhibitors. In total, we identified 43 essential effector genes to be linked to the RNAi pathway of T. canis ( Supplementary Data 13 ), complementing the information for nematodes [42] . Compared with A. suum , we found the genes pash-1 and rde-4 , encoding small RNA biosynthetic proteins, as well as the nuclear RNAi effector gene ekl-1 in T. canis . However, we detected neither the RNAi inhibitor nor the effector genes adr-2 and gfl-1 , respectively, in this nematode. We identified a full repertoire of genes encoding argonautes, including nrde-3 . The genes encoding small interfering RNA amplification effectors as well as dsRNA uptake and spreading factors were consistent with those in A. suum [42] , except sid-1 which is present in T. canis . All of the effectors identified were transcribed in the gut and tissues of adult females and males of T. canis . Argonautes were particularly highly transcribed in adult worms compared with third-stage larvae (L3). The apparent absence of the sid-2 gene suggests that the uptake of extracellular dsRNA is compromised [43] . Some evidence indicating that gene knock-down can be achieved in larvae of A. suum [44] , [45] shows promise for functionality testing of conserved and also orphan (‘parasite-specific’) genes in T. canis larvae. Following extensive work, compounds rationally designed to selected targets could be tested and assessed in vivo in experimentally infected animals (for example, dogs or mice). High throughput nucleic acid sequencing and bioinformatic approaches are having far-reaching implications for investigating socioeconomically important parasites. The present genomic and transcriptomic exploration provides a global insight into the molecular biology of T. canis , a zoonotic parasite of major animal and human health importance worldwide. We predicted molecules involved in host–parasite interactions and immune responses, and studied transcriptional differences between two stages and sexes, as well as the gut of the adult stage of the parasite. The present draft genome and transcriptomes of T. canis should accelerate post-genomic explorations. For instance, a systems biology-based approach should now facilitate many aspects of the developmental and reproductive biology, molecular biology and biochemistry of T. canis , as well as parasite–host interactions and the pathogenesis of toxocariasis to be explored, also based on the knowledge of homologs/orthologs and information in curated, public databases. The characterization of the RNAi machinery in of T. canis could provide a solid platform for fundamental, functional genomic work in selected stages (for example, cultured larvae) of the parasite. Technological advances also provide prospects for large-scale investigations of the proteome and metabolome of T. canis . In addition, the use of advanced glycomic methods [46] should provide profound insights into the often heavily glycosylated proteins in Toxocara ES products [5] , [23] , [24] . Clearly, the present genome and transcriptomic data provide the critical resources to enable the transition from ‘single-molecule’ research to global molecular discovery in T. canis . This exciting prospect could lead to a paradigm shift in our understanding of this enigmatic parasite and to significant advances in applied areas, including the development of drugs, vaccines and diagnostic tests. Although this study focused on T. canis , the findings and the technological approaches used should be readily applicable to a wide range of other ascaridoid nematodes of major animal and human health importance. Procurement of T. canis Fresh specimens of T. canis (adults) expelled from a naturally infected domestic dog and faeces from the same, infected dog were given to one of us (P.N.) by a dog owner from Næstved, Denmark. Worms and eggs were identified morphologically [47] . Eggs were isolated from the faeces by sieving (mesh sizes: 500, 200, 90 and then 60 μm) and purified by sugar-salt flotation [48] , washed in water and then allowed to fully embryonate in H 2 SO 4 (pH 2.0) at 22 °C for 30 days. L3s were released from within their egg shells by glass-bead (400 μm) beating for 40 min (37 °C), concentrated for 3 h at 37 °C in 5% CO 2 in a Baermann funnel [49] ; then, L3s were washed extensively in sterile saline, pelleted and snap-frozen in liquid nitrogen. Adult stages of T. canis were washed extensively in saline (37 °C), sexes separated and then snap-frozen individually and stored at −80 °C until use; the specific identity of each specimen was verified by PCR-based sequencing of the second internal-transcribed spacer of nuclear ribosomal DNA (NCBI accession identifier Y09489) [50] . Genomic DNA, library construction and sequencing High molecular weight genomic DNA was isolated from a single immature adult male of T. canis using a commercial kit (Chemagic STAR DNA Tissue Kit, Perkin Elmer) according to the manufacturer’s protocol. The DNA yield was measured spectrophotometrically (Qubit fluorometer dsDNA HS Kit, Invitrogen); DNA integrity was verified by agarose-gel electrophoresis and using a Bioanalyzer (2100, Agilent). Paired-end (PE) genomic libraries (with 170-, 500- and 800-bp inserts) as well as jumping (J) genomic libraries (with 2-, 5-, and 10-kb inserts) were constructed according to manufacturer’s instructions (Illumina); to produce sufficient amounts of DNA for these latter libraries, 250–500 ng of genomic DNA were subjected to whole-genome amplification using the REPLI-g midi kit (Qiagen), as recommended. All sequencing was carried out on GA II or HiSeq (Illumina; 2 × 75 or 2 × 100 reads for paired-end libraries, and 2 × 49 reads for J-libraries), and reads were exported to the FASTQ format. RNA isolation and RNA-seq RNA was isolated separately from different developmental stages and body parts of T. canis (three biological replicates of L3s; and four replicates of each female and male reproductive tracts; female and male anterior bodies; female and male guts) employing TriPure (Roche Molecular Biochemicals). For L3s, packed volumes of 20–50 μl were used, equating to thousands of larvae. For other stages and components, packed volumes of 100–200 μl from single worms were used. RNA yields were estimated spectrophotometrically (NanoDrop 1000), and integrity was verified using a Bioanalyzer. RNA-seq was carried out according to manufacturer’s instructions (Illumina). Pre-processing of sequence reads Genomic and RNA-seq reads derived from individual libraries were assessed for quality, adaptors removed and sequencing errors corrected using an in-house pipeline. Then, any dog ( Canis lupus familiaris ; host of T. canis ) and bacterial sequences were identified by comparison with the sequences in the ENSEMBL (release 72) and NCBI (8 April 2013) databases, respectively. In brief, all libraries were aligned to the Canis lupus familiaris genome using SOAPaligner v.2.21 ( http://soap.genomics.org.cn/soapaligner.html ) and reads that mapped to the genome removed. To remove bacterial sequences, one million randomly selected reads per library were aligned (≥80% of read length and ≥90% sequence identity in overlapping regions) to known bacterial genomes using BLAST v.2.2.26; low complexity reads were not aligned. Transcriptome assembly Pre-processed RNA-seq reads were assembled de novo using the program Trinity (v.r2012-06-08) [51] and also employing a genome-guided approach employing the programs TopHat2 v.2.0.7 (ref. 52 ) and Cufflinks2 v.2.1.1 (ref. 53 ). First, to achieve a consensus (non-redundant) set of transcripts, the open reading frames (ORFs) of all transcripts were predicted. Second, a single transcript with the longest ORF was retained, if another transcript mapped to the same exon in the reference genome and shared the same reading frame, and if the length of the exonic (coding) regions covered by both transcripts divided by length of the shortest ORF was >30%. Both genome-guided and de novo -assembled transcriptomes for individual stages and tissues of T. canis were used for the prediction of genes. Genome assembly Pre-processed genomic PE-libraries (insert sizes 170-, 500- and 800-bp) and J-libraries (insert sizes: 2-, 5 -and 10-kb) were assembled and scaffolded using the program SOAPdenovo2 v.2.04 ( http://soap.genomics.org.cn/soapdenovo.html ) using a k-mer of 43. The GapCloser v.1.10 program within the SOAPdenovo2 suite was used to close gaps in the scaffolded assembly. The completeness of the T. canis draft genome assembly was estimated using the program CEGMA and the number of core eukaryotic genes [54] . Prediction of repetitive elements First, repeat sequences were masked using the programs LTR_FINDER v.1.0.5 (ref. 55 ), PILER v.1.0 (ref. 56 ), RepeatScout v.1.0.5 (ref. 57 ), RepeatMasker v.open-4.0.3 (ref. 58 ) and Tandem Repeat Finder v.4.07 (ref. 59 ) using a collection of known repeats in Repbase v.17.02 (ref. 60 ). Then, all transposons were combined and a non-redundant set of representative transposons produced by selecting the longest transposon (representing each subclass) that overlapped in sequence by >30% with the shortest transposon. Identification and annotation of non-coding regions and protein-coding genes The T. canis protein-coding genes were predicted de novo from the repeat-masked draft genome and also using homology- and RNA-seq-based approaches against the unmasked genome. The predictions were then merged into a non-redundant gene set using the program GLEAN [61] . The training gene set for the de novo predictions was inferred from transcriptomes assembled using the program Cuffmerge v.2.1.1 (ref. 53 ). First, for each locus with multiple transcripts, only the longest ORF was retained. Second, protein sequences inferred from the longest ORFs in the resultant, non-redundant data set were aligned to the NCBI nr database (released on 4 September 2013) using the program BLASTp. Matches that aligned over >80% of their length both in reference and query and had >75% identity represented the training set for the de novo gene-prediction programs AUGUSTUS [62] , GlimmerHMM [63] and SNAP [64] . Using each of these programs, a gene set was predicted de novo from the assembled draft genome. In addition, RNA-seq-, EST- and homology-based gene sets were predicted, which were then, together with de novo -predictions, subjected to analysis using the program GLEAN to infer a reference set of genes for T. canis . UTR-regions were removed from RNA-seq-based, genome-guided and de novo -assembled transcriptomes using an in-house pipeline. The prediction of the EST data set of T. canis was aided by the NCBI EST database (8 September 2014) using the program BLASTn v.2.2.26. Homology-based comparisons were made with the proteomes of A. suum , B. malayi , C. elegans and P. pacificus . The reference gene set of T. canis was refined by using gene-prediction models supported by (i) both homology and RNA-seq evidence (>20 mapped reads); (ii) homology-based models only, with no frame-shift mutations and an alignment length of ≥50% of the query sequence; and (iii) RNA-seq models only, but encoding proteins of ≥120 amino acids in length. UTRs from RNA-seq data were added to the gene predictions using TopHat2 v.2.0.7. Finally, genes inferred to encode peptides of ≥50 amino acids were preserved; genes predicted were represented by their coding and inferred amino acid sequences. Functional annotation of all predicted protein sequences First, following the prediction of the protein-coding gene set for T. canis , each inferred amino acid sequence was assessed for conserved protein domains using InterProScan 5 Web Services ( http://www.ebi.ac.uk/Tools/pfa/iprscan5/ ) and InterPro 44.0 ( http://www.ebi.ac.uk/interpro/ ). Second, amino acid sequences were subjected to BLASTp v.2.2.26 (E-value≤10 −8 ) using the following protein databases: C. elegans in WormBase WS240 ( www.wormbase.org ); Swiss-Prot and TrEMBL (released in March 2013) within UniProtKB; (KEGG release 58); NCBI protein nr (released in September 2013). On the basis of the KEGG BLAST matches, the KEGG BRITE hierarchy was used to classify predicted proteins into families; each coding gene was assessed against the known KO-term BLAST matches using a custom script; these matches were collected to known protein families in KEGG BRITE defined in the KEGG Orthology Based Annotation System database. ES proteins were predicted using the programs Phobius ( http://www.ebi.ac.uk/Tools/pfa/phobius/ ), SignalP ( http://www.cbs.dtu.dk/services/SignalP/ ) and TMHMM ( http://www.cbs.dtu.dk/services/TMHMM/ ). The predicted proteins were listed, as were their annotations based on the conserved InterProScan domain matches with respective gene ontology terms and then (successively) based on their homology matches (E-value cut-off: ≤10 −8 ) to proteins in: the Swiss-Prot, C. elegans , the KEGG, NCBI nr and TrEMBL databases. Any predicted protein without a match (E-value cut-off: ≤10 −8 ) in at least one of these databases was designated an hypothetical protein. The final annotation for the protein-coding gene set of T. canis is available for download at http://bioinfosecond.vet.unimelb.edu.au/Tcanis . Structural modelling was conducted using the program Phyre ( http://www.sbg.bio.ic.ac.uk/phyre2/ ). RNAi pathway prediction The RNAi effectors were predicted by the program BLAST v2.2.28 (E-value≤10 −15 ) using internal protein database and a database of effector sequences [42] . Predictions were verified against the final functional annotations for T. canis and with the inferred proteome of A. suum (WormBase; WS230). For each gene, levels of transcription in different developmental stages and tissues (gut and reproductive) were normalized using the trimmed mean of M-values scale-normalization method [65] . Differential transcription analysis and integrated enrichment The analysis of RNA-seq data representing different developmental stages, body parts and genders of T. canis was conducted using the program edgeR ( http://www.bioconductor.org/packages/release/bioc/html/edgeR.html ). Individual pre-processed PE RNA-seq data sets (three replicates) were mapped to the predicted gene set using TopHat2 v.2.0.7. The numbers of reads that mapped to each gene were enumerated using the program SAMtools [66] . For each replicate of each data set (sample), the resultant read counts were used as input data for edgeR. The levels of differential transcription were calculated based on pairwise comparisons among samples of T. canis (that is, L3 versus female anterior; L3 versus male anterior; female anterior versus female reproductive tract; male anterior versus male reproductive tract; female reproductive tract versus male reproductive tract; female anterior versus female gut; male anterior versus male gut; female gut versus male gut). Using dispersion factors calculated in edgeR, the genes were considered differentially transcribed if the fold change compared with the normalized read count data was ≥2, and the false discovery rate was ≤0.05. In addition, enrichment clusters of significantly differentially transcribed genes were defined (Fisher’s exact test) and an integrated analysis was conducted. Using a custom script, data linked to these gene clusters were enriched from KEGG pathway and KEGG BRITE hierarchy database. Hubs of these gene clusters were identified using functional gene networking ( C. elegans ; http://geneorienteer.org/ ) and weighted gene co-expression network analysis [67] , [68] . Orthology First, orthologs were predicted by pairwise comparison of individual proteins (predicted from each gene set) among T. canis , A. suum , B. malayi , C. elegans and P. pacificus using the OrthoMCL v.1.4 (ref. 69 ) and BLASTp (cut-off: 10 −5 ). Results obtained using these two approaches were displayed in a Venn diagram. Prediction of essential molecules Essential genes/gene products were predicted [70] , but using reciprocal best BLAST hits to infer orthologous groups. Lethal phenotypes (WBPhenotype:0000062 and sub-phenotypes (listed in http://www.berkeleybop.org/ontologies/wbphenotype.obo ) in C. elegans were identified in WormBase WS240. Network connectivity data for C. elegans were obtained using WormNet v.2 ( http://www.functionalnet.org/wormnet/cgi-perl/WormNet.v2_nga_form.cgi ). Additional analyses, and use of software for document preparation We conducted analyses in a Unix environment or Microsoft Excel 2007 using standard commands. Bioinformatic scripts required to facilitate data analysis were designed using mainly the Python2.6 scripting language and are available via http://research.vet.unimelb.edu.au/gasserlab/ . How to cite this article : Zhu, X.-Q. et al . Genetic blueprint of the zoonotic pathogen Toxocara canis . Nat. Commun. 6:6145 doi: 10.1038/ncomms7145 (2015). Accession codes: Sequence data are accessible via National Center for Biotechnology Information (NCBI; www.ncbi.nlm.nih.gov ) under accession code JPKZ00000000 (version JPKZ00000000.1; GI:734563511; BioProject: PRJNA248777 ).